Negative electrostatic potentials in a Hofmann-type metal-organic framework for efficient acetylene separation Efficient adsorptive separation of acetylene (C 2 H 2 ) from carbon dioxide (CO 2 ) or ethylene (C 2 H 4 ) is industrially important but challenging due to the identical dynamic diameter or the trace amount. Here we show an electrostatic potential compatible strategy in a nitroprusside-based Hofmann-type metal-organic framework, Cu(bpy)NP (NP = nitroprusside, bpy = 4,4’-bipyridine), for efficient C 2 H 2 separation. The intruding cyanide and nitrosyl groups in undulating one-dimensional channels induce negative electrostatic potentials for preferential C 2 H 2 recognition instead of open metal sites in traditional Hofmann-type MOFs. As a result, Cu(bpy)NP exhibits a 50/50 C 2 H 2 /CO 2 selectivity of 47.2, outperforming most rigid MOFs. The dynamic breakthrough experiment demonstrates a 99.9% purity C 2 H 4 productivity of 20.57 mmol g −1 from C 2 H 2 /C 2 H 4 (1/99, v / v ) gas-mixture. Meanwhile, C 2 H 2 can also be captured and recognized from ternary C 2 H 2 /CO 2 /C 2 H 4 (25/25/50, v/v/v ) gas-mixture. Furthermore, computational studies and in-situ infrared spectroscopy reveal that the selective C 2 H 2 binding arises from the compatible pore electro-environment generated by the electron-rich N and O atoms from nitroprusside anions. Acetylene (C 2 H 2 ) capture from gas-mixtures is of great industrial importance [1] , [2] . As a vital chemical feedstock and industrial gas [3] , C 2 H 2 is typically generated by the partial combustion of methane, a considerable amount of carbon dioxide (CO 2 ) inevitably coexists in the crude products. 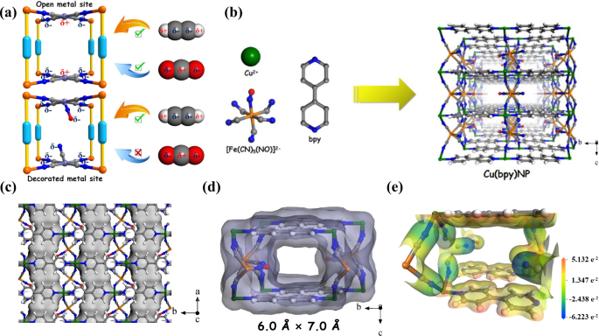Fig. 1: Material synthesis and crystallographic structures. Schematic illustration ofatraditional and nitroprusside-based Hofmann-type MOF networks andbthe building blocks (Cu2+, [Fe(CN)5(NO)]2−, and bpy) and the 3Dsqc-net topology of Cu(bpy)NP;cview of the pore channels by the Connolly surface along theab-plane,dillustration of the channel size along thebc-plane, andethe ESP mapping for the channel of Cu(bpy)NP (color code: C, gray; H, white; N, blue; O, red; Cu, green; Fe, orange). C 2 H 2 and CO 2 molecules both possess linear configurations with subtle differences in molecular dimensions (3.3 × 3.3 × 5.7 Å for C 2 H 2 and 3.2 × 3.3 × 5.4 Å for CO 2 ), and show close similarities in physical properties, including quadrupole moments, boiling point, and polarity (Supplementary Table 1 ) [4] , [5] . On the other hand, the highly reactive C 2 H 2 can induce undesirable side effects in various industrial operations. For instance, in ethylene (C 2 H 4 ) manufacturing by the steam cracking of naphtha or dehydrogenation of ethane [6] , [7] , the trace amount of C 2 H 2 (1%) must be removed to an acceptable level of 40 ppm, otherwise the residue C 2 H 2 will deactivate the Ziegler–Natta catalyst and lower the quality of polyethylene commodities [8] . In industry, trace C 2 H 2 removal is achieved by partial hydrogenation or solvent absorption, which are energy- and cost-intensive [9] . Therefore, alternative technologies with high capital efficiency have attracted great interest in separating C 2 H 2 from CO 2 and C 2 H 4 due to their industrial relevance and scientific challenge, such as adsorptive separations [10] . Since the discovery of Prussian blue in 1704, transition metal cyanide complexes, also referred to as cyanometallates, have been extensively synthesized [11] . The strong basicity of cyanide, as δ -donor and π -acceptor, endows the ability and versatility of coordination with most transition metals [12] . Particularly, cyanide-based metal-organic frameworks (MOFs) with interior vacancies and open spaces emerge as an intriguing class of solid adsorbents [13] , [14] . As a family of Prussian blue analogs, Hofmann-type MOFs have a general formula of M(pyz)[M’(CN)] 4 , where M and M’ are divalent metal ions and pyz is the pyrazine bidentate organic ligand [15] . Besides the confined pore spaces, another prevailing feature is the existence of abundant open metal sites (OMSs) incorporated in cyanometallate ligand that can significantly enhance the C 2 H 2 capacity through strong electrostatic interactions. For example, Co(pyz)[Ni(CN)] 4 , termed as ZJU-74a, exhibited the record C 2 H 2 adsorption capacity of 49 cm 3 g −1 at 0.01 bar and 296 K due to the sandwich-like open Ni sites from adjacent [Ni(CN)] 4 2− ligands [13] . However, the open Ni sites can also interact with the electronegative O atoms of CO 2 (Fig. 1a ), as evidenced by the close C 2 H 2 and CO 2 capacity (3.82 mmol g −1 vs 3.13 mmol g −1 ) at 1.0 bar and 296 K. Fig. 1: Material synthesis and crystallographic structures. Schematic illustration of a traditional and nitroprusside-based Hofmann-type MOF networks and b the building blocks (Cu 2+ , [Fe(CN) 5 (NO)] 2− , and bpy) and the 3D sqc -net topology of Cu(bpy)NP; c view of the pore channels by the Connolly surface along the ab -plane, d illustration of the channel size along the bc -plane, and e the ESP mapping for the channel of Cu(bpy)NP (color code: C, gray; H, white; N, blue; O, red; Cu, green; Fe, orange). Full size image Nitroprusside is a unique type of cyanide ligand in which the Fe(II) atoms are octahedrally coordinated by five carbon atoms from independent cyanide groups and one nitrogen atom from a nitrosyl group (Fig. 1b ). The straightforward coordination of Cd 2+ and Ni 2+ ions with nitroprusside (NP) have yielded Cd-NP and Ni-NP that showed superior CO 2 /C 2 H 2 and C 3 H 6 /C 3 H 8 separation performances [11] , [16] , respectively. Nevertheless, to the best of our knowledge, the successful preparation of Hofmann-type MOFs using nitroprusside ligand has never been reported. Unlike the directly exposed OMSs in cyanometallate ligand, the intruding cyanide and nitrosyl groups can create a negative-charged electrostatic potential field for preferred C 2 H 2 capture, because C 2 H 2 possesses a positive charge distribution at both ends (Fig. 1a ) [14] . Note that creating a negative-charged pore environment is challenging due to the limited choice of suitable functional groups. Herein, we report a Hofmann-type MOFs employing nitroprusside ligand, Cu(bpy)NP (NP = nitroprusside, bpy = 4,4’-bipyridine), for efficient and selective capture of C 2 H 2 from C 2 H 2 /CO 2 and C 2 H 2 /C 2 H 4 gas-mixtures. In particular, Cu(bpy)NP exhibits a three-dimensional sqc topology with a suitable cavity size of 6.0 × 7.0 Å 2 . The incorporation of cyanide and nitrosyl groups on the pore walls afford a complementary negative electrostatic potential field for C 2 H 2 binding. As a result, Cu(bpy)NP shows a large C 2 H 2 capacity (50.7 cm 3 g −1 ) and superior C 2 H 2 /CO 2 (47.2) and C 2 H 2 /C 2 H 4 (28.5) selectivity at 298 K and 1.0 bar. Dynamic breakthrough experiments confirm its practical C 2 H 2 capture performances from binary C 2 H 2 /CO 2 and C 2 H 2 /C 2 H 4 gas-mixtures and ternary C 2 H 2 /CO 2 /C 2 H 4 gas-mixture. Cu(bpy)NP affords C 2 H 4 productivity of 20.57 mmol g −1 from C 2 H 2 /C 2 H 4 (1/99, v/v ) gas-mixture. Theoretical modeling and in-situ IR studies reveal that C 2 H 2 molecules are collectively bound by two nitrosyl groups and one cyanide group via multiple strong interactions. Synthesis and characterization By dripping the aqueous solution of Cu(NO 3 ) 2 ·3H 2 O and sodium nitroprusside (NP) into a methanol solution of 4,4’-bipyridine (bpy), the Cu(bpy)NP can be obtained under mild conditions with a yield of 67% (Fig. 1b ). Cyan square-block single-crystals of Cu(bpy)NP were also successfully prepared by the slow-diffusion method (Supplementary Fig. 1 ). Single-crystal X-ray diffraction studies revealed that Cu(bpy)NP crystallizes in an orthorhombic space group Pmma and adopts a 4,6-connected sqc topology (Fig. 1b , CCDC: 2124121). Each Cu moiety is octahedrally coordinated by two ditopic bridging bpy linkers at the axial positions and four independent cyanide groups from [Fe(CN) 5 (NO)] 2− anions at equatorial positions (Supplementary Fig. 2 ). In the structure of Cu(bpy)NP, the undulating two-dimensional (2D) channels across the ab -plane are different from the regular one-dimensional (1D) channels in previously reported Hofmann-type MOFs (Fig. 1c ) [12] , [13] . The channels in Cu(bpy)NP showed a channel dimension of 6.0 × 7.0 Å 2 along the bc -plane (Fig. 1d ). The volume of its solvent-accessible void was calculated to be 34.4% of the total volume. Moreover, the electrostatic potential (ESP) of channel interior in Cu(bpy)NP was mapped by density functional theory (DFT) calculations (Fig. 1e ), and strong negative potentials were disclosed near the nitrogen atom in the cyanide group and oxygen atom in the nitrosyl group that are compatible for C 2 H 2 adsorption, however, which are mutually repulsive to CO 2 with negatively charged ends (Supplementary Fig. 3 ). The phase purity of the as-synthesized Cu(bpy)NP was verified by the powder X-ray diffraction (PXRD) pattern, which is consistent with the simulated one, while no noticeable change was observed on the activated sample (Supplementary Fig. 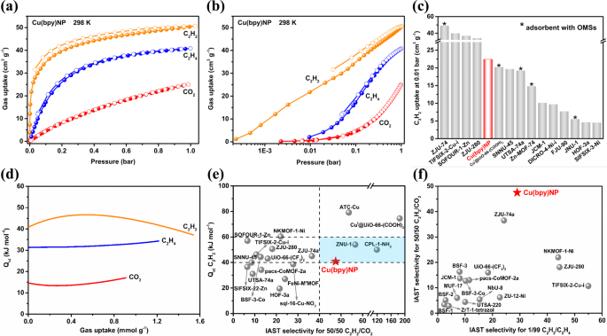Fig. 2: C2H2, CO2, and C2H4sorption in nitroprusside-based Hofmann-type MOFs. C2H2, CO2, and C2H4adsorption isothermsain linear form andbin logarithmic form of Cu(bpy)NP at 298 K;ccomparison of C2H2uptakes with best-performing materials at 0.01 bar and 298 K;dQstplots of C2H2, CO2, and C2H4on Cu(bpy)NP;ecomparison of C2H2Qstand 50/50 C2H2/CO2IAST selectivity with leading adsorbents;fcomparison of 50/50 C2H2/CO2and 1/99 C2H2/C2H4IAST selectivity of Cu(bpy)NP with reported adsorbents at 298 K and 1.0 bar. 4 Supplementary Table 2 ). Furthermore, the Rietveld refinement of PXRD revealed that the activated Cu(bpy)NP crystallized in the same crystal system and showed similar cell parameters with the as-synthesized sample, indicating its rigid framework after solvent removal (Supplementary Fig. 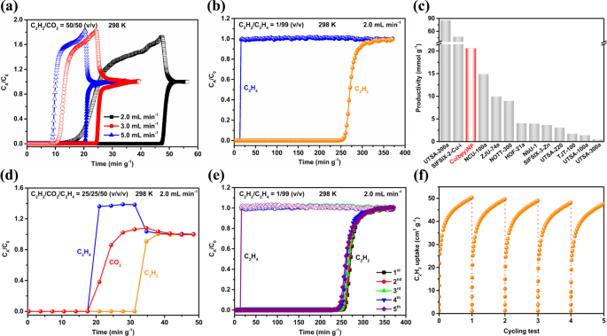Fig. 3: C2H2, CO2, and C2H4separation performances. Dynamic breakthrough curves of Cu(bpy)NP foraC2H2/CO2(50/50,v/v) andbC2H2/C2H4(1/99,v/v) gas-mixtures;ccomparison of C2H4productivity with representative MOFs;ddynamic breakthrough curve of Cu(bpy)NP for ternary C2H2/CO2/C2H4(25/25/50,v/v/v) gas-mixture;ecycling dynamic breakthrough tests for C2H2/C2H4(1/99,v/v) on Cu(bpy)NP;fcontinuous five C2H2adsorption isotherms of Cu(bpy)NP at 298 K. 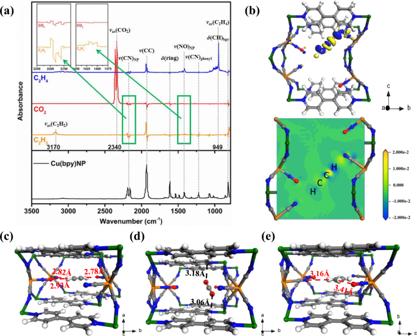Fig. 4: In-situ IR spectra and binding sites for C2H2, CO2, and C2H4in Cu(bpy)NP. aIn-situ IR spectra of gas-loaded Cu(bpy)NP samples;bCharge density difference plots showing the interaction between C2H2; DFT-D calculated binding sites ofcC2H2,dCO2, andeC2H4in Cu(bpy)NP. The distances include the Van der Waals radius of atoms (Color code: C, gray; H, white; N, blue; O, red; Cu, green; Fe, orange). 5 and Supplementary Table 3 ). The PXRD patterns of C 2 H 2 -loaded samples under different pressures (0–1.0 bar) at 298 K showed inconspicuous changes in position and intensity of diffraction peaks, manifesting structural robustness during adsorption processes (Supplementary Fig. 6 ). The structural integrity was examined by immersing Cu(bpy)NP in various organic solvents for 1 week and boiling water for 3 h, intact PXRD patterns can be maintained, suggesting its good chemical stability (Supplementary Fig. 7a ). Meanwhile, Cu(bpy)NP could survive wide range acid/basic solutions, whereas the crystal structure was destroyed at extreme conditions, i.e., pH = 13 and 1 (Supplementary Fig. 7b ). TGA revealed a weight loss of 2.9% at 220 °C, corresponding to the removal of guest molecules (Supplementary Fig. 8 ). The Brunauer-Emmett-Teller (BET) surface area of Cu(bpy)NP was measured to be 459 m 2 g −1 with a total pore volume of 0.45 cm 3 g −1 by CO 2 adsorption at 195 K (Supplementary Fig. 9 ). The pore size was determined to center at 6.6 Å, consistent with the channel size derived from the crystal structure. The pore properties were also probed by N 2 at 77 K (Supplementary Fig. 10 ), the decreased BET specific surface area of 121 m 2 g −1 can be attributed to the larger size and property inertness of N 2 as the probe molecule. Adsorption and separation performances Single-component gas adsorption isotherms of C 2 H 2 , CO 2 , and C 2 H 4 were collected at 273, 298, and 323 K, respectively (Fig. 2a , Supplementary Fig. 11 , and Supplementary Tables 6 - 8 ). Cu(bpy)NP exhibited a higher C 2 H 2 adsorption capacity (50.7 cm 3 g −1 ) than that of C 2 H 4 (40.8 cm 3 g −1 ) and CO 2 (25.1 cm 3 g −1 ) at 298 K and 1.0 bar. Approximately, two C 2 H 2 , one CO 2 , and one and a half C 2 H 4 molecules are adsorbed per unit cell, respectively. Generally, the gas separation performances greatly correlate with the gas adsorption behaviors in low-pressure ranges, in which the adsorbent-adsorbate affinity dominates [17] . As shown in Fig. 2b , Cu(bpy)NP displayed a C 2 H 2 uptake of 22.4 cm 3 g −1 at 0.01 bar and 298 K, notably, even comparable to adsorbents with OMSs, including Cu I @UiO-66-(COOH) 2 (20.2 cm 3 g −1 ) [18] , UTSA-74a (19.2 cm 3 g −1 ) [19] , Zn-MOF-74 (14.8 cm 3 g −1 ) [20] , and JNU-1 (5.5 cm 3 g −1 ) [21] (Fig. 2c and Supplementary Table 9 ). In sharp contrast, the adsorption uptake of C 2 H 4 (2.1 cm 3 g −1 ) and CO 2 (0.6 cm 3 g −1 ) was almost negligible at 0.01 bar. The adsorption isotherms have experimentally confirmed the concept that the negative electrostatic potential can selectively adsorb C 2 H 2 over CO 2 and C 2 H 4 . Fig. 2: C 2 H 2 , CO 2 , and C 2 H 4 sorption in nitroprusside-based Hofmann-type MOFs. C 2 H 2 , CO 2 , and C 2 H 4 adsorption isotherms a in linear form and b in logarithmic form of Cu(bpy)NP at 298 K; c comparison of C 2 H 2 uptakes with best-performing materials at 0.01 bar and 298 K; d Q st plots of C 2 H 2 , CO 2 , and C 2 H 4 on Cu(bpy)NP; e comparison of C 2 H 2 Q st and 50/50 C 2 H 2 /CO 2 IAST selectivity with leading adsorbents; f comparison of 50/50 C 2 H 2 /CO 2 and 1/99 C 2 H 2 /C 2 H 4 IAST selectivity of Cu(bpy)NP with reported adsorbents at 298 K and 1.0 bar. Full size image To evaluate the affinity of Cu(bpy)NP toward C 2 H 2 , CO 2 , and C 2 H 4 , the isosteric enthalpy of adsorption ( Q st ) was calculated by Virial fitting from adsorption isotherms at three temperatures (Supplementary Fig. 12 and Supplementary Table 10 ). The calculated Q st for C 2 H 2 is 40.8 kJ mol −1 , higher than that of CO 2 (14.6 kJ mol −1 ) and C 2 H 4 (31.3 kJ mol −1 ) at near zero coverage (Fig. 2d ). The moderate Q st for C 2 H 2 indicates both strong binding and energy-efficient regeneration (Fig. 2e ) [22] . Moreover, the difference in Q st (Δ Q st ) represents the binding selectivity of adsorbents, the Δ Q st for C 2 H 2 and CO 2 is calculated to be 26.2 kJ mol −1 , which is the most prominent except for two MOFs with rich OMSs (Supplementary Fig. 17 ), i.e., Cu I @UiO-66-(COOH) 2 (45.6) [18] and ATC-Cu (42.6) [23] . The ideal adsorbed solution theory (IAST) was employed to evaluate the adsorptive separation selectivity, and the adsorption isotherm fittings by the dual-site Langmuir-Freundlich model were shown in Supplementary Figs. 13 – 15 and Supplementary Table 11 . First, the adsorption kinetics of C 2 H 2 , CO 2 , and C 2 H 4 were evaluated on Cu(bpy)NP, which depicted that the equilibrium times for all gases were about 6 min at 298 K and 0.4 bar (Supplementary Fig. 16 ). Benefiting from the preferred C 2 H 2 adsorptions at low pressures, Cu(bpy)NP exhibited a benchmark 50/50 C 2 H 2 /CO 2 selectivity of 343.8 at 0.01 bar and 298 K, and gradually decreased to 47.2 at 1.0 bar (Supplementary Fig. 18 ). Notably, such C 2 H 2 /CO 2 selectivity at ambient conditions, to our knowledge, is only lower than benchmark adsorbents such as Cu I @UiO-66-(COOH) 2 (185) [18] , CPL-1-NH 2 (119) [24] , ZNU-1 (56.6) [25] , and ATC-Cu (53.6) [24] , and higher than leading materials including ZJU-74a (36.5) [13] , NKMOF-1-Ni (22.0) [17] , and HOF-3a (21.5) [26] (Fig. 2e ). It is worth pointing out that Cu(bpy)NP should be considered as one of the most promising candidates that show favorable C 2 H 2 /CO 2 selectivity (>40) and suitable C 2 H 2 Q st for regeneration (40~60 kJ mol −1 ) [22] . Similarly, the 1/99 C 2 H 2 /C 2 H 4 IAST selectivity of 781.2 and 28.5 was obtained at 0.01 bar and 1.0 bar and 298 K, respectively (Supplementary Fig. 19a ). Besides the advantageous C 2 H 2 /C 2 H 4 IAST selectivity (Supplementary Fig. 19b and Supplementary Table 9 ), noticeably, the C 2 H 2 /CO 2 IAST selectivity on Cu(bpy)NP was also superior to many reported adsorbents (Fig. 2f ). Transient breakthrough experiments To further experimentally validate the separation performances of Cu(bpy)NP, dynamic breakthrough experiments were carried out under ambient conditions. As shown in Fig. 3a , Cu(bpy)NP can efficiently separate an equimolar gas-mixture of C 2 H 2 /CO 2 , at a flow rate of 2.0 mL min −1 , CO 2 was detected first at the outlet of the separation bed at around 20 min, while C 2 H 2 was not eluted from the column until 78 min. The separation selectivity ( α AC ) for equimolar C 2 H 2 /CO 2 mixture was calculated to be 3.9 on Cu(bpy)NP based on the breakthrough curve, outperforming SNNU-45 (2.9) [27] , NKMOF-1-Ni (2.6) [17] , HOF-3a (2.0) [27] , and FeNi-M’MOF (1.7) [14] (Supplementary Fig. 20 ). When the flow rate increased to 3.0 and 5.0 mL min −1 , the breakthrough time decreased as expected but good separation effects remained. Meanwhile, as illustrated by the desorption curves, CO 2 desorbed quickly in 10 min and the complete desorption of C 2 H 2 was achieved at 90 min, indicating a long operation window for C 2 H 2 collection with high C 2 H 2 purity above 99% (Supplementary Fig. 21 ). As for C 2 H 2 /C 2 H 4 (1/99, v/v ) gas-mixture, C 2 H 4 immediately broke through the packed column with Cu(bpy)NP at 22 min, while C 2 H 2 was trapped and eluted until 400 min (Fig. 3b ). The C 2 H 4 productivity with 99.9 + % purity was calculated to be 20.57 mmol g −1 on Cu(bpy)NP, which is only lower than that of SIFSIX-2-Cu-i (47.4 mmol g −1 ) [9] and UTSA-200a (85.7 mmol g −1 ) [28] (Fig. 3c ). Even when the concentration of C 2 H 2 increased to 50%, Cu(bpy)NP also maintained the efficient and clean separation for C 2 H 2 /C 2 H 4 (50/50, v/v ) gas-mixture (Supplementary Fig. 22 ). Fig. 3: C 2 H 2 , CO 2 , and C 2 H 4 separation performances. Dynamic breakthrough curves of Cu(bpy)NP for a C 2 H 2 /CO 2 (50/50, v/v ) and b C 2 H 2 /C 2 H 4 (1/99, v/v ) gas-mixtures; c comparison of C 2 H 4 productivity with representative MOFs; d dynamic breakthrough curve of Cu(bpy)NP for ternary C 2 H 2 /CO 2 /C 2 H 4 (25/25/50, v/v/v ) gas-mixture; e cycling dynamic breakthrough tests for C 2 H 2 /C 2 H 4 (1/99, v/v ) on Cu(bpy)NP; f continuous five C 2 H 2 adsorption isotherms of Cu(bpy)NP at 298 K. Full size image Furthermore, we also carried out the dynamic breakthrough experiment with ternary C 2 H 2 /CO 2 /C 2 H 4 (25/25/50, v/v/v ) gas-mixture. As shown in Fig. 3d , CO 2 and C 2 H 4 concurrently broke through the adsorption column at 28 min, whereas C 2 H 2 was not detected at the exit until 50 min. The cycling and regeneration capabilities of Cu(bpy)NP are important parameters for practical industrial applications. Therefore, cycling breakthrough cycle experiments for both C 2 H 2 /CO 2 (50/50, v/v ) and C 2 H 2 /C 2 H 4 (1/99, v/v ) were conducted (Fig. 3e and Supplementary Fig. 23 ), during five continuous cycles, no noticeable decay in the residual time was observed. Also, five successive C 2 H 2 adsorption-desorption isotherms showed intact C 2 H 2 uptakes, manifesting the excellent reusability of Cu(bpy)NP (Fig. 3f ). In-situ IR and modeling simulation studies In-situ infrared (IR) spectroscopic measurements were conducted on gas-loaded samples to illustrate the interactions between three adsorbates and Cu(bpy)NP. It is recognized that acidic C 2 H 2 molecules tend to form strong interactions with basic sites [8] , [29] . As shown in Fig. 4a , the ν as (C 2 H 2 ) stretching band of adsorbed C 2 H 2 down-shifted to 3170 cm −1 with reference to the gas-phase value at 3287 cm −1 , indicating the existence of guest–host interactions with possible charge transfers [30] , [31] , [32] . The strong perturbation of characteristic bands, i.e., ν(CN) NP , ν (CC) bpy , ν (CN) bpy , δ (CH) bpy , ν (NO) NP , and δ (ring), suggested that C 2 H 2 also interacted with Cu(bpy)NP framework via multiple weak interactions. The adsorbed CO 2 within Cu(bpy)NP was confirmed by its asymmetric stretching band ν as (CO 2 ) at 2340 cm −1 [33] . Compared to the C 2 H 2 -loaded framework, the perturbations of characteristic bands were obviously decreased in intensity, especially for ν (CN) NP and ν (NO) NP (Fig. 4a inset), verifying that the complementary electrostatic potential created by cyanide and nitrosyl groups were responsible for selective C 2 H 2 capture. As for C 2 H 4 , the ν as (C 2 H 4 ) stretching band appeared at 949 cm −1 [34] , [35] , and the interaction mode was similar to that of C 2 H 2 -loaded samples. It was noted that the ν (NO) NP bond was intensified, indicating the favorable affinity toward nitrosyl groups. Fig. 4: In-situ IR spectra and binding sites for C 2 H 2 , CO 2 , and C 2 H 4 in Cu(bpy)NP. a In-situ IR spectra of gas-loaded Cu(bpy)NP samples; b Charge density difference plots showing the interaction between C 2 H 2 ; DFT-D calculated binding sites of c C 2 H 2 , d CO 2 , and e C 2 H 4 in Cu(bpy)NP. The distances include the Van der Waals radius of atoms (Color code: C, gray; H, white; N, blue; O, red; Cu, green; Fe, orange). Full size image To gain insight into the adsorption mechanisms of C 2 H 2 , CO 2 , and C 2 H 4 in Cu(bpy)NP, theoretical molecular simulations using the grand canonical Monte Carlo (GCMC) and first-principles dispersion-corrected density functional theory (DFT-D) were carried out. The GCMC-simulated C 2 H 2 , CO 2 , and C 2 H 4 adsorption isotherms agreed well with the experimental isotherms (Supplementary Fig. 24 ). The distribution densities were firstly investigated at 1 kPa, C 2 H 2 molecules are mainly distributed in two locations near the cyanide and nitrosyl groups. In sharp contrast, the CO 2 molecules are distributed in the middle of the channels that are apart from nitroprusside anions. Whereas, the C 2 H 4 molecules occupy almost identical locations in the channels of Cu(bpy)NP but with less distribution density compared to C 2 H 2 (Supplementary Fig. 25a–c ). As the loading pressure increased to 100 kPa, the adsorption locations for each adsorbent remained, while the contribution density is in the order of C 2 H 2 > C 2 H 4 > CO 2 , which is consistent with the experimental adsorption capacities (Supplementary Fig. 25d–f ). We firstly carried out the charge transfer analysis on the gas-loaded structures by DFT calculations. As shown in Fig. 4b , the blue and yellow surfaces indicate charge accumulation and charge depletion, respectively. The close end-on adsorption configuration of H atom of C 2 H 2 and N atom of cyanide groups implied the strong electro-field induced C 2 H 2 capture (Fig. 4b ). Moreover, the negatively charged H atom of C 2 H 2 , opposite to its original positive-charged state, revealed the charge transfer from Cu(bpy)NP framework to adsorbed C 2 H 2 . In contrast, CO 2 and C 2 H 4 molecules displayed the side-on adsorption configurations in Cu(bpy)NP skeleton, and no noticeable charge transfer was observed (Supplementary Fig. 26 ). These results highlighted the effect of negatively charged pore environment in enhancing the adsorption and recognition of C 2 H 2 . The lowest-energy gas binding configurations of C 2 H 2 , CO 2 , and C 2 H 4 in Cu(bpy)NP were also calculated. As shown in Fig. 4c , C 2 H 2 was roughly oriented parallel to the bpy ligand along the a -axis, where it was captured by three independent [Fe(CN) 5 (NO)] 2− anions via strong interactions of two C-H•••O bonds (2.78–2.93 Å) and one C-H•••N bond (2.82 Å). The binding energy of C 2 H 2 in Cu(bpy)NP was calculated to be 38.4 kJ mol −1 , slightly lower than the experimental C 2 H 2 Q st (40.8 kJ mol −1 ). In contrast, CO 2 was adsorbed by two opposite bpy ligands through weak interactions of N•••O(CO 2 ) (3.06 Å) and C•••C(CO 2 ) (3.18 Å) with a calculated CO 2 binding energy of 13.4 kJ mol −1 (Fig. 4d ). Clearly, the negative electrostatic potential generated by [Fe(CN) 5 (NO)] 2− anions induced the preferential binding with C 2 H 2 over CO 2 . Similarly, Cu(bpy)NP displayed relatively weak interactions with C 2 H 4 via the C-H•••N bond (3.16 Å) and C-H•••O bond (3.41 Å), the C 2 H 4 binding energy was calculated to be 28.5 kJ mol −1 (Fig. 4e ). In summary, we synthesized and reported a nitroprusside-based Hofmann-type MOF adsorbent, Cu(bpy)NP, for simultaneous efficient separation of C 2 H 2 from C 2 H 2 /CO 2 and C 2 H 2 /C 2 H 4 gas-mixtures. Compared to the traditional Hofmann-type MOFs with rich OMSs, the cyanide and nitrosyl groups of nitroprusside anions generated a negative electro-environment in the undulating 1D channels for the preferential discrimination of C 2 H 2 over CO 2 . Consequently, Cu(bpy)NP exhibited a high 50/50 C 2 H 2 /CO 2 selectivity and 1/99 C 2 H 2 /C 2 H 4 selectivity. A considerable balance of separation selectivity and adsorption enthalpy was achieved on Cu(bpy)NP. Dynamic breakthrough experiments revealed the advantageous C 2 H 4 productivity with 99.9% purity. Modeling studies and in-situ IR measurements indicated the compatible pore environment and strong guest-host interactions for efficient C 2 H 2 separation. This work encourages the community to design and synthesize Hofmann-type adsorbents for challenging separation tasks. All reagents were purchased from commercial companies and used without further purification. Sodium nitroprusside dihydrate (C 5 FeN 6 Na 2 O·2H 2 O, 99.98%, Aladdin), copper nitrate trihydrate (Cu(NO 3 ) 2 ·3H 2 O, 99.99%, Aldrich), 4,4’-bipyridine (C 10 H 8 N 2 , 98%, Aladdin), and methanol (CH 4 O, anhydrous, 99.9%, Aladdin) were commercially available and used as supplied without further purification. N 2 (99.999%), acetylene (C 2 H 2 , 99.99%), CO 2 (99.99%), ethylene (C 2 H 4 , 99.99%), He (99.999%), and mixed gas-mixtures of C 2 H 2 /CO 2 (50/50, v/v ), C 2 H 2 /C 2 H 4 (1/99, v/v ), C 2 H 2 /C 2 H 4 (50/50, v/v ), and C 2 H 2 /CO 2 /C 2 H 4 (25/25/50, v/v/v ) were purchased from Nanchang Guoteng Gas Co., Ltd (China). Synthesis of Cu(bpy)NP Typically, Cu(NO 3 ) 2 ·3H 2 O (0.25 mmol, 60 mg) and sodium nitroprusside (NP, 0.25 mmol, 75 mg) were dissolved in 3 mL H 2 O and then dripped into a methanol solution (30 mL) of 4,4’-bipyridine (bpy, 0.2 mmol, 35 mg) under vigorous stirring. After reacting at room temperature in the dark for 48 h, cyan precipitates were collected by centrifugation, washed thrice with methanol, and dried overnight in a vacuum oven at 333 K (yield: ca . 67% based on NP). Single-crystals of Cu(bpy)NP were synthesized by slow diffusion of a methanol solution (0.4 mL) of NP (0.003 mmol, 0.89 mg) and bpy (0.002 mmol, 0.35 mg) into an aqueous solution (0.4 mL) of Cu(NO 3 ) 2 ·3H 2 O (0.003 mmol, 0.72 mg) at room temperature in the dark in a watch glass and kept undisturbed, and 1.2 mL of methanol/H 2 O (1:1) was layered between the top and bottom solutions to slow the reaction rate. Light cyan and square prismatic crystals were formed after 1 week. Structure simulations The unit cell structures (e.g., cell parameters and atomic positions) of Cu(bpy)NP were calculated using the Forcite and Castep modules. The Rietveld refinement, a software package for crystal determination from the XRD pattern, was performed to optimize the lattice parameters iteratively until the w R p value converges. The pseudo-Voigt profile function was used for whole profile fitting, and the Berrar-Baldinozzi function was used for asymmetry correction during the refinement processes. Line broadening from crystallite size and lattice strain were both considered. Gas adsorption measurements Equilibrium and kinetic adsorptions of C 2 H 2 , CO 2 , and C 2 H 4 at 273, 298, and 323 K were measured on Micromeritics ASAP 2460 adsorption apparatus (Micromeritics Instruments, USA). The kinetic adsorptions of C 2 H 2 , CO 2 , and C 2 H 4 were obtained on Intelligent Gravimetric Analyzer (IGA-100, HIDEN). To remove all the guest solvents in the framework, the fresh powder samples were evacuated under a high vacuum at 373 K for 12 h. The BET surface area was calculated using the adsorption branch with the relative pressure P/P 0 range of 0.005–0.3. The total pore volume (V tot ) was calculated based on the adsorbed amount of nitrogen at the P/P 0 of 0.99. The pore size distribution (PSD) was calculated based on CO 2 and N 2 adsorption isotherms at 195 K and 77 K, respectively. The helium gas was used to determine the free space of the system. The sample was degassed for 24 h between each measurement. In-situ infrared (IR) spectroscopic measurements All the IR spectroscopic data are recorded in a Tensor 27 FTIR spectrometer (Bruker, GER) equipped with a liquid N 2 -cooled mercury cadmium telluride MCT-A detector. A vacuum cell, purchased from Specac Ltd., UK (product number P/N 5850c), is placed in the sample compartment of the infrared spectrometer with the sample at the beam’s focal point. The cell is connected to different gas lines (C 2 H 2 , CO 2 , and C 2 H 4 ) and a vacuum line for evacuation. The Cu(bpy)NP (powder, ~30 mg) was placed in the cell, and firstly annealed at 100 °C under vacuum for activation and then cooled to RT for recording the reference spectrum. C 2 H 2 was introduced into the cell, and the spectra were recorded during the gas exposure till 60 min. After fully evacuating the same sample by pumping the cell, the reference spectrum was retaken. Loading of CO 2 and C 2 H 4 was performed separately, and the infrared data were recorded in the same manner. Breakthrough experiments The breakthrough experiments were performed on a self-assembly device. Typically, the activated Cu(bpy)NP (about 1.65 g) was packed into a stainless-steel column (4.6 mm inner diameter × 100 mm). The column was first purged with a He flow (10 mL min −1 ) at room temperature for 8 h before breakthrough measurements. The binary C 2 H 2 /CO 2 (50/50, v/v ), C 2 H 2 /C 2 H 4 (1/99, v/v ), and ternary C 2 H 2 /CO 2 /C 2 H 4 (25/25/50, v/v/v ) gas-mixtures were then introduced at a flow rate of 2.0, 3.0, and 5.0 mL min −1 , respectively. The outlet gas from the column was monitored using gas chromatography (GC-490 plus) with a flame ionization detector. After the breakthrough measurement, the columns packed with samples were regenerated by purging dry He gas (10 mL min −1 ) at 100 °C for 24 h. DFT calculations First-principles DFT calculations were performed using Materials Studio’s CASTEP code. All calculations were conducted under the generalized gradient approximation (GGA) with Perdew-Burke-Ernzerhof (PBE). The optimized structures are in great consistency with the experimentally determined crystal structures. The energy, force, and displacement convergence criteria were set as 1 × 10 −5 Ha, 2 × 10 −3 Ha, and 5 × 10 −3 Å, respectively. Single point energy calculations with the same parameters using Dmol 3 were performed on optimized Cu(bpy)NP. The electron density data obtained from these calculations were used to construct the 0.015 e − Å −3 electron density isosurfaces of the C 2 H 2 and CO 2 molecules, while the electron density data of both frameworks were used to construct the 0.15 e − Å −3 electron density isosurfaces, with a grid interval of 0.1 Å. The calculated electrostatic potential for Cu(bpy)NP and C 2 H 2 and CO 2 molecules were then mapped onto their electron density isosurfaces. A semiempirical addition of dispersive forces to conventional DFT was included in the calculation to account for van der Waals interactions. Cutoff energy of 544 eV and a 2 × 2 × 2 k-point mesh were enough for the total energy coverage within 0.01 meV atom −1 . The structures of the synthesized materials were first optimized from the reported crystal structures. The pristine structure and an isolated gas molecule placed in a supercell (with the same cell dimensions as the pristine crystal structure) were optimized and relaxed as references to obtain the binding energy. C 2 H 2 , CO 2 , and C 2 H 4 gas molecules were then introduced to different locations of the channel pore, followed by a full structural relaxation. The static binding energy was calculated by the equation E B = E (gas) + E (adsorbent) − E (adsorbent + gas). GCMC calculations All the GCMC simulations were performed in MS 2017R2 package. The crystal structure of the Cu(bpy)NP was chosen after the DFT geometry optimization. The framework and the individual C 2 H 2 , CO 2 , and C 2 H 4 were considered rigid during the simulation. The charges for atoms of the Cu(bpy)NP and gas components were derived from the Muliken method. The simulations adopted the fixed pressure task, the Metropolis method in the sorption module, and the universal force field (UFF). The interaction energy between the adsorbed molecules and the framework was computed through the Coulomb and Lennard–Jones 6-12 (LJ) potentials. The cutoff radius was chosen 18.5 Å for LJ potential and the electrostatic interactions were handled using the Ewald summation method. The loading and equilibration steps were 1 × 10 7 , and the production steps were 1 × 10 7 . Sample characterizations PXRD was collected on a PANalytical Empyrean Series 2 diffractometer with Cu Kα radiation ( λ = 1.540598 Å), which operated at 40 kV, 40 mA, and a scan speed of 0.0167°, a scan time of 15 s per step, and 2θ ranging from 5 to 60° at room temperature. The thermogravimetric analysis (TGA) data were performed on a NETZSCH Thermogravimetric Analyzer (STA2500) from 25 to 800 °C with a heating rate of 10 °C/min under an N 2 atmosphere. The single-component adsorption isotherms of C 2 H 2 , CO 2 , and C 2 H 4 at 273, 298, and 323 K were measured on Micromeritics ASAP 2460 adsorption apparatus (Micromeritics Instruments, USA). The degassing procedure for all samples was carried out at 373 K under vacuum for 12 h before each adsorption measurement. The specific BET surface area was calculated based on the CO 2 adsorption isotherm data (0.05 and 0.15 relative pressure) at 195 K. The PSD was derived from the adsorption branch of CO 2 isotherms using the non-local density functional theory method and assuming a slit pore model. Single-crystal X-ray diffraction Single-crystal X-ray diffraction data for Cu(bpy)NP were collected at 193(2) K on a Bruker-AXS D8 VENTURE diffractometer equipped with a PHOTON-100/CMOS detector (GaKα, λ = 1.3414 Å). Indexing was performed using APEX2. SaintPlus 6.01 was used to complete data integration and reduction. The multi-scan method implemented in SADABS was used to conduct absorption correction. XPREP implemented in APEX2.1 was used to determine the space group. The structures were solved by direct methods and refined by nonlinear least-squares on the F2 method with SHELXL-97 contained in APEX2, OLEX2 v1.1.5, and WinGX v1.70.01 program packages. The Squeeze routine implemented in Platon was used to treat the contribution of disordered solvent molecules as diffuse. Crystallographic data are available free of charge from the Cambridge Crystallographic Data Center (CCDC). The CCDC number for the Cu(bpy)NP crystal is 2124121. Structural stability tests Solvent stability tests were performed by placing 100 mg samples in 20 mL vials containing 15 mL of different organic solvents for 1 week, boiling water for 3 h, and acid/basic solutions with different pH for 1 week. Then, the solid was separated by filtration and subsequently activated at 100 °C for 12 h, and PXRD tests characterized the structure of the materials. Fitting of isotherms The single-component isotherms for C 2 H 2 , CO 2 , and C 2 H 4 on Cu(bpy)NP were fitted with the dual-site Langmuir-Freundlich isotherm model: 
    q=q_1b_1p^v_1/1+b_1p^v_1+q_2b_2p^v_2/1+b_2p^v_2
 (1) with T-dependent parameters b 
    b=b_0exp(E/RT)
 (2) Where q is the adsorbed amount for an adsorbent in mmol g −1 , q 1 , q 2 is the saturated adsorption capacities in mmol g −1 , b is the Langmuir parameters in kPa −1 , p is pressure in kPa −1 , ν is the Freundlich parameters for single-sites, R is the gas constant, and T (K) is the temperature. The model fits the pure component isotherms well, and the R 2 values are more significant than 0.9994 (see Table S6 ). IAST calculations of adsorption selectivity IAST calculations of adsorption selectivity for C 2 H 2 /CO 2 and C 2 H 2 /C 2 H 4 separation was defined by 
    S_ads=q_1/q_2/p_1/p_2
 (3) q 1 and q 2 are the molar loadings in the adsorbed phase in equilibrium with the bulk gas phase, p 1 and p 2 are partial pressures. Separation factor/separation selectivity calculations The amount of adsorbed gas i ( q i ) is calculated from the breakthrough curve as follows: 
    q_i=V_iT_0- V_dead-∫_0^t_0V_e T/m
 (4) Here, V i is the influent flow rate of gas (cm 3 min −1 ), V e is the effluent flow rate of gas (cm 3 min −1 ), V dead is the dead volume of the system (cm 3 ), t is the adsorption time (min) and m is the mass of the sorbent ( g ) [1] . On approximation, this simplifies to: 
    q_i=V_TTP_i/m
 (5) V T is the total flow rate of gas (cm 3 min −1 ), P i is the partial pressure of gas i (bar) and ΔT is the time for the initial breakthrough of gas i to occur (min) [2] . The separation factor, also known as separation selectivity ( α AC ) for the breakthrough experiment, i.e., breakthrough-derived selectivity is determined as follows: 
    α=q_1 y_2/q_2 y_1
 (6) y i is the partial pressure of gas i in the gas-mixture. If one gas component has negligible adsorption, the amount of gas adsorbed is treated as ≤1 cm 3 for calculations. Isosteric heat of adsorption The binding energies of C 2 H 2 , CO 2 , and C 2 H 4 are reflected indirectly in the isosteric heat of adsorption, Q st , which are calculated by the Clausius-Clapeyron equation, defined as 
    Q_st=-RT^2(∂lnP/∂lnT)n_a
 (7) where Q st represents the adsorption heat of C 2 H 2 , C 2 H 4 , and CO 2 , P , and T represent the pressure and temperature under adsorption measurement conditions, and R is the universal gas constant. Here, the adsorption heat of each component was determined precisely according to the virial fitting parameters of single-component adsorption isotherms measured at 273, 298, and 323 K up to 1.0 bar, which was defined as follows: 
    InP=In N+1/T ∑_i=0^ma_iN^i + ∑_i=0^nb_iN^i
 (8) 
    Q_st=-R∑_i=0^ma_iN_i
 (9) where the N is the adsorption amount, and m and n determine the number of items required to precisely fit the adsorption isotherms.